A new class of plant lipid is essential for protection against phosphorus depletion Phosphorus supply is a major factor responsible for reduced crop yields. As a result, plants utilize various adaptive mechanisms against phosphorus depletion, including lipid remodelling. Here we report the involvement of a novel plant lipid, glucuronosyldiacylglycerol, against phosphorus depletion. Lipidomic analysis of Arabidopsis plants cultured in phosphorus-depleted conditions revealed inducible accumulation of glucuronosyldiacylglycerol. Investigation using a series of sulfolipid sulfoquinovosyldiacylglycerol synthesis-deficient mutants of Arabidopsis determined that the biosynthesis of glucuronosyldiacylglycerol shares the pathway of sulfoquinovosyldiacylglycerol synthesis in chloroplasts. Under phosphorus-depleted conditions, the Arabidopsis sqd2 mutant, which does not accumulate either sulfoquinovosyldiacylglycerol or glucuronosyldiacylglycerol, was the most severely damaged of three sulfoquinovosyldiacylglycerol-deficient mutants. As glucuronosyldiacylglycerol is still present in the other two mutants, this result indicates that glucuronosyldiacylglycerol has a role in the protection of plants against phosphorus limitation stress. Glucuronosyldiacylglycerol was also found in rice, and its concentration increased significantly following phosphorus limitation, suggesting a shared physiological significance of this novel lipid against phosphorus depletion in plants. Phosphorus (P) is an essential component in cells and has a crucial role in cellular functionality and metabolism. However, because of limited P availability in many soils, plants often suffer from P deficiency [1] . Indeed, it is estimated that crop yields for 40% of the world’s arable land are reduced because of P unavailability [2] . As current known P reserves are limited and P-based fertilizers are economically produced, efficient use and the minimization of the loss of P resources (that is, recycling of struvite, magnesium ammonium phosphate) are very important to sustainable agriculture [3] , [4] , [5] . However, plants have developed several adaptation mechanisms to cope with P-limited environments. P mobilization by membrane lipid remodelling, that is, changing the composition of the membrane lipids rich in phospholipids, is one of the general mechanisms of adapting to P limitation in plants [6] , [7] , [8] , [9] . Replacement of membrane phospholipids with non-phosphorus glycerolipids such as sulfoquinovosyldiacylglycerol (SQDG) and digalactosyldiacylglycerol (DGDG), which promote the remobilization of P, is typical of metabolic signatures associated with lipid remodelling during phosphate deprivation. These glycolipids are usually found in chloroplast membranes, but DGDG is also found in extraplastidic membranes in P-starved plants [7] , [8] , [10] . Thus far, various aspects of lipid remodelling following P limitation have been investigated. The biosynthetic enzymes involved in the enhanced production of these non-phosphorus glycolipids under P limitation, mainly glycosyltransferases and sugar-donor synthetic enzymes, have been intensely characterized [11] , [12] , [13] , [14] , [15] , [16] , [17] , [18] . Phospholipid degradation and P recycling have also been analysed through the characterization of several phospholipases and glycerophosphodiesterases [15] , [19] , [20] , [21] , [22] . In addition, parts of the signal transduction pathway for lipid remodelling have been studied [14] , [15] , [23] , [24] . However, detailed metabolite analysis regarding lipid remodelling has been limited. Previous studies have thus far focused only on several well-known lipid classes [25] because of the difficulties associated with the comprehensive analysis of plant lipids, which consist of a wide variety of hydrophobic chemicals. In this study, we applied untargeted metabolomic analysis, which allows comprehensive chemical metabolic phenotyping of cells, to investigate lipid remodelling in detail and to identify a new key lipid molecule that has an essential role in protection against P-depletion stress. A new plant lipid inducibly accumulates under P depletion To expose plants to P-limiting stress, wild-type Arabidopsis thaliana plants grown on phosphate (P i )-sufficient growth medium for 14 days were transferred to either P i -sufficient or P i -depleted growth medium. After another 14 days of growth, lipids were extracted from the leaves and subjected to lipidomic analysis by hydrophilic interaction chromatography (HILIC) coupled with ion trap time-of-flight mass spectrometry [26] . This analysis indicated that P limitation induced a decrease in phospholipids such as phosphatidylglycerol (PG), phosphatidylethanolamine (PE), phosphatidylinositol (PI) and phosphatidylcholine, with a complementary increase in non-phosphorus glycerolipids, including SQDG (~4.5-fold) and DGDG (~2-fold), as previously reported ( Fig. 1a ) [7] , [12] . The total monogalactosyldiacylglycerol (MGDG) level did not significantly change in response to P limitation, as described below ( Fig. 1a ). In addition to these changes, a new peak (UK1; retention time, 11.4 min) was found to appear under P limitation but not under P sufficiency. To obtain detailed information regarding the overall metabolic changes induced by P limitation, an orthogonal projection to a latent structure-discriminant analysis (OPLS-DA) model was examined using the lipidomic data obtained from the plants subjected to P-limited and P-sufficient conditions [27] . The OPLS-DA ( Supplementary Fig. S1 ) and OPLS loading S-plot ( Fig. 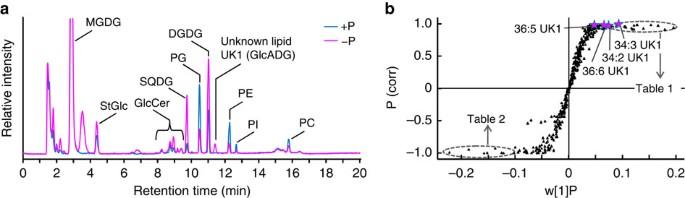Figure 1: A new lipid inducibly accumulates inArabidopsisunder P depletion. (a) Wild-typeArabidopsisplants grown under P-sufficient conditions were transferred to either P-sufficient (+P, blue line) or P-depleted (−P, red line) medium. After cultivation for 14 days, crude lipid extracts from the leaves were analysed by HILIC-MS. The total ion current detected by the negative ion mode is shown. An unknown lipid (denoted as UK1, further identified as GlcADG) appeared only under P-limited conditions. (b) S-plot of OPLS-DA based on ANOVA of the cross-validated residuals (CV-ANOVA). The S-plot demonstrates the covariance versus the correlation in conjunction with the variable trend plots and allows easier visualization of the data. The variables that showed maximum change, and therefore strongly contributed to the class separation, are plotted at the top or bottom of the S-shaped plot. The variables that did not significantly vary are plotted in the middle. Each point represents a lipid molecule detected in the negative ion mode. Red stars denote the [M–H]−ions of the UK1 species, indicating that the change in the levels of a series of UK1 molecules is highly associated with P-limiting treatment. The molecules at the top and bottom are listed inTables 1and2. 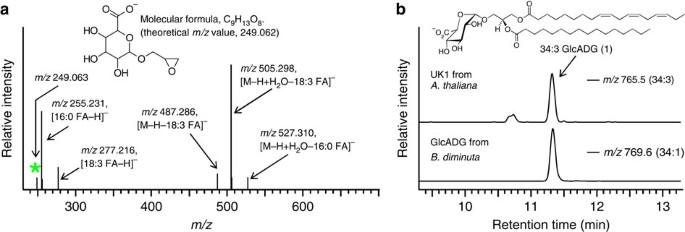Figure 2: The novel lipid is glucuronosyldiacylglycerol (GlcADG). (a) MS/MS of [M–H]−ion of the major UK1 molecule (34:3 UK1.m/z765.517). FA, fatty acid. The asterisk indicates the key fragment ion attributable to the glucuronosylglycerol moiety. (b) Comparison of the chromatographic behaviour of UK1 and GlcADG isolated fromB. diminuta. The structure of the most major GlcADG molecule fromArabidopsis(34:3 GlcADG) is presented. The species labels, namely, total acyl carbons:total acyl double bonds, are shown in parentheses. Fragment analysis in the negative mode allowed annotation of fatty acyl groups and tentative assignment of these groups to thesn-1 andsn-2 positions60. 1b ) revealed that the discriminative inducible metabolites associated with the P-limiting treatment were mainly UK1, SQDG and DGDG ( Table 1 ), and the significantly decreased metabolites were phospholipids ( Table 2 ). We focused on the new lipid UK1 for further study. Figure 1: A new lipid inducibly accumulates in Arabidopsis under P depletion. ( a ) Wild-type Arabidopsis plants grown under P-sufficient conditions were transferred to either P-sufficient (+P, blue line) or P-depleted (−P, red line) medium. After cultivation for 14 days, crude lipid extracts from the leaves were analysed by HILIC-MS. The total ion current detected by the negative ion mode is shown. An unknown lipid (denoted as UK1, further identified as GlcADG) appeared only under P-limited conditions. ( b ) S-plot of OPLS-DA based on ANOVA of the cross-validated residuals (CV-ANOVA). The S-plot demonstrates the covariance versus the correlation in conjunction with the variable trend plots and allows easier visualization of the data. The variables that showed maximum change, and therefore strongly contributed to the class separation, are plotted at the top or bottom of the S-shaped plot. The variables that did not significantly vary are plotted in the middle. Each point represents a lipid molecule detected in the negative ion mode. Red stars denote the [M–H] − ions of the UK1 species, indicating that the change in the levels of a series of UK1 molecules is highly associated with P-limiting treatment. The molecules at the top and bottom are listed in Tables 1 and 2 . Full size image Table 1 Discriminative metabolites predicted by OPLS-DA with increased levels following P deprivation. Full size table Table 2 Discriminative metabolites predicted by OPLS-DA with decreased levels following P deprivation. Full size table Mass spectral analyses revealed that UK1 is a lipid class consisting of several similar molecular species whose molecular weights differed by 2 Da ( Supplementary Fig. S2a,c ). The tandem mass spectrum (MS/MS) of UK1 further revealed that the major product ions were attributable to two fatty acids and glucuronosylglycerol ( Fig. 2a , and Supplementary Fig. S2b ), which suggests that UK1 is a glucuronosylated diacylglycerol ( Fig. 2b ). MS/MS results in the positive ion mode, exhibiting the neutral loss attributable to glucuronic acid, also supported this conclusion ( Supplementary Fig. S2c,d ). The presence of 1,2-diacyl-3- O -α-glucuronosylglycerol (GlcADG, 1 ) has been reported in several bacteria and fungi and in two species of unicellular algae [28] , [29] , [30] , but it has not yet been described in higher plants. In addition, the physiological function and biosynthetic gene have not been identified in these organisms. Thus, we purified UK1 from A. thaliana and GlcADG from the proteobacterium Brevundimonas diminuta , previously called Pseudomonas diminuta [31] , and compared them with respect to several physicochemical properties. Figure 2: The novel lipid is glucuronosyldiacylglycerol (GlcADG). ( a ) MS/MS of [M–H] − ion of the major UK1 molecule (34:3 UK1. m/z 765.517). FA, fatty acid. The asterisk indicates the key fragment ion attributable to the glucuronosylglycerol moiety. ( b ) Comparison of the chromatographic behaviour of UK1 and GlcADG isolated from B. diminuta . The structure of the most major GlcADG molecule from Arabidopsis (34:3 GlcADG) is presented. The species labels, namely, total acyl carbons:total acyl double bonds, are shown in parentheses. Fragment analysis in the negative mode allowed annotation of fatty acyl groups and tentative assignment of these groups to the sn -1 and sn -2 positions [60] . Full size image The new plant lipid was identified as GlcADG The purified UK1 and bacterial GlcADG showed the same chromatographic behaviour ( Fig. 2b ) and same fragmentation pattern ( Fig. 2a , and Supplementary Figs S3,S4 ), supporting the hypothesis that UK1 was GlcADG. However, further characterization of the sugar moiety was still required to identify UK1. At first, we intended to analyse the NMR spectra of UK1 using bacterial GlcADG as the reference; however, NMR spectra of GlcADG from B. diminuta were not available because the bacterial GlcADG was identified via several other methods of chemical derivatization [31] . Thus, we carefully analysed the structure of these two lipids from two different organisms. First, GlcADG from B. diminuta was hydrolysed with hydrochloric acid, and the hydrolysate was analysed using GC–MS. The compound found in the hydrolysate was identified as glucuronic acid, not galacturonic acid, by comparison with the commercially available standard ( Supplementary Figs S5,S6 ), indicating that the glycosyl moiety of isolated bacterial lipid is glucuronic acid. Then, we analysed NMR spectra of the methyl ester of GlcADG from B. diminuta . The 1 H and 13 C NMR data on the methyl ester of bacterial GlcADG is very similar to previously published data on GlcADG from Caulobacter bacteroides [32] and Aspergillus fumigates [33] , respectively, considering the effect of methylation of the carboxyl group of glucuronic acid. In addition, the 1 H and 13 C NMR spectra of the methyl ester of UK1 are also very similar to those of the methyl ester of bacterial GlcADG. Thus, the lipids isolated from A. thaliana and B. diminuta are both GlcADG ( 1 ). The coupling constants of the anomeric proton (H-1′) of GlcADG from A. thaliana and B. diminuta are both 3.7 Hz, indicating that the configuration of the glycosidic bond in these lipids is ‘alpha’. The coupling pattern of protons in the uronic acid moiety is also consistent with the conclusion that the sugar moiety of this lipid class is glucuronic acid. Elucidation of the possible biosynthetic pathway of GlcADG The biosynthesis of lipids occurs in the discrete subcellular biogenic membranes of different cellular compartments, and the fatty composition of the glycerolipids synthesized in one compartment is quite different from those synthesized in other compartments. For example, endoplasmic reticulum-derived glycerolipids have an 18-carbon fatty acid at sn- 2 of glycerol, while glycerolipids synthesized de novo in plastids have a 16-carbon fatty acid at sn- 2 (refs 34 , 35 ). Some of these lipids are transported from one compartment to another and transformed into different lipid classes by changing their polar headgroup. This transformation is catalysed by several different enzymes that are not evenly distributed in every organelle. These mechanisms for membrane lipid biosynthesis make the fatty acid composition and diacylglycerol (DAG) composition of each lipid class unique. Thus, the MS and MS/MS spectral information obtained as lipidomic data were further utilized to elucidate the biosynthetic mechanism of GlcADG production, based on the assumption that each glycerolipid class possesses a characteristic fatty acid composition that reflects their synthetic route. Hierarchical clustering (HCL) of the z -scored DAG composition of each lipid class demonstrated that the DAG composition of GlcADG and SQDG were nearly identical, indicating that GlcADG belongs to the same group as the SQDG produced during P limitation ( Fig. 3a ). Analysis of the negative MS/MS data on these lipids further confirmed the high similarities between the fatty acid compositions of GlcADG and SQDG ( Supplementary Fig. S3 ). It should be noted that all plant GlcADG species with acyl groups consisting of 34 carbons have a palmitic acid moiety at the sn -2 position ( Supplementary Fig. S3 ). Palmitic acid (16:0 fatty acid) is a minor acyl group both in galactolipids and at sn -2 of phospholipids, but it is the major group at sn -2 in SQDG ( Supplementary Fig. S3 ) [34] , [35] . These results collectively suggest that the biosynthesis of GlcADG may share, at least in part, the biosynthetic pathway of SQDG. 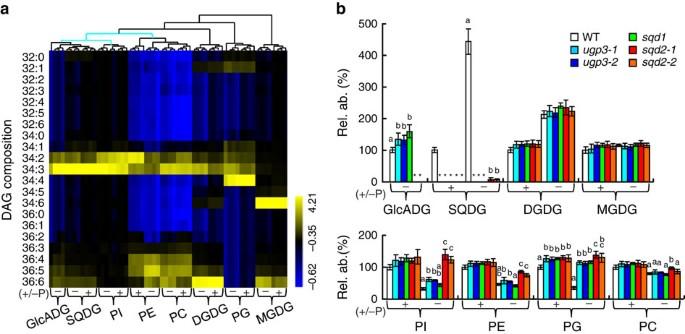Figure 3: Compositional changes of lipid species under P starvation. (a) HCL of glycerolipid classes based on thez-scored DAG compositions of the fatty acid moieties.Key: P-sufficient (+P), P-depleted (−P). To test the rigour of the presented dendrogram, we performed a permutation test using jackknife resampling (permutation, 1,000). The colours of the branches indicate the level of branch rearrangement reliability (jackknife proportions) (black: 95–100% support, blue: 80–90% support). (b) Levels of individual lipid classes are expressed as relative abundance (Rel. ab.) against that of the wild-type grown under P-sufficient conditions. GlcADG was not detected under the P-sufficient condition. Each data point represents the mean±s.d. value of four experiments. Different letters indicate statistically significant differences (P<0.05, Tukey’s test) among the tested genotypes grown under identical growth conditions. The absence of letters demonstrates no significant difference among all the tested genotypes for a lipid class. The asterisk denotes ‘not detected’. Figure 3: Compositional changes of lipid species under P starvation. ( a ) HCL of glycerolipid classes based on the z -scored DAG compositions of the fatty acid moieties. Key : P-sufficient (+P), P-depleted (−P). To test the rigour of the presented dendrogram, we performed a permutation test using jackknife resampling (permutation, 1,000). The colours of the branches indicate the level of branch rearrangement reliability (jackknife proportions) (black: 95–100% support, blue: 80–90% support). ( b ) Levels of individual lipid classes are expressed as relative abundance (Rel. ab.) against that of the wild-type grown under P-sufficient conditions. GlcADG was not detected under the P-sufficient condition. Each data point represents the mean±s.d. value of four experiments. Different letters indicate statistically significant differences ( P <0.05, Tukey’s test) among the tested genotypes grown under identical growth conditions. The absence of letters demonstrates no significant difference among all the tested genotypes for a lipid class. The asterisk denotes ‘not detected’. Full size image SQDG synthase is required for GlcADG synthesis In A. thaliana , SQDG is synthesized in the chloroplast by three unique steps ( Fig. 4a ): synthesis of UDP-glucose (UDP-Glc) by UDP-Glc pyrophosphorylase 3 (UGP3) [17] , assembly of UDP-Glc and sulphite into UDP-sulfoquinovose (UDP-SQ) by UDP-SQ synthase (SQD1) [11] , [36] , and the subsequent transfer of the SQ moiety from UDP-SQ to DAG by SQDG synthase (SQD2) [12] , [37] . These three SQDG biosynthetic enzymes are located in the chloroplast, and the expression of their coding genes is coordinated in green tissues and significantly upregulated by P limitation [11] , [12] , [17] , [37] , [38] , [39] , [40] . Based on the above-mentioned hypothesis that GlcADG synthesis partly shares the pathway of SQDG synthesis, GlcADG accumulation was investigated in a series of mutants deficient in all three SQDG biosynthetic genes of A. thaliana under the P-depleted condition. The sqd1 and ugp3 mutants produced GlcADG at a slightly higher level than the wild-type control ( Fig. 3b and Supplementary Fig. S7 ); strikingly, however, no accumulation of GlcADG was observed in the independent sqd2 mutants. These results clearly demonstrate that GlcADG is synthesized by the action of SQD2 ( Fig. 4a ), presumably using DAG and a sugar donor—most likely UDP-glucuronic acid (UDP-GlcA)—instead of UDP-SQ, which is used in the synthesis of SQDG. However, two other enzymes involved in SQDG synthesis, UGP3 and SQD1, are not involved in the synthesis of GlcADG. 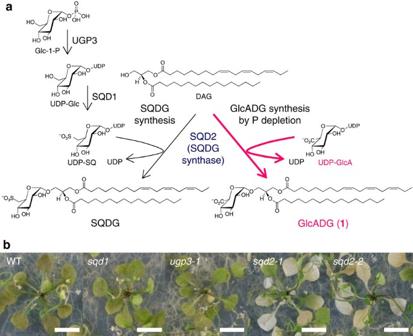Figure 4: Investigation of GlcADG biosynthesis and growth phenotypes ofArabidopsismutants. (a) Three enzymes (UGP3, SQD1 and SQD2) are involved in the biosynthesis of SQDG in the chloroplasts ofArabidopsis. SQD2 is responsible for SQDG synthesis under P-sufficient conditions. Under P-deficient conditions, SQD2 produces not only SQDG but also GlcADG. (b) Wild-type plants and a series of SQDG-deficient mutants ofA. thalianagrown under P-sufficient conditions were transferred to either P-sufficient or P-depleted medium. After cultivation for 4 weeks, the growth of each genotype was compared. The individuals showing the most typical phenotype of P deprivation are displayed. Only 2sqd2mutants appeared bleached under P-starvation conditions. Scale bar, 1 cm. Images of other individuals are shown inSupplementary Fig. S11. Figure 4: Investigation of GlcADG biosynthesis and growth phenotypes of Arabidopsis mutants. ( a ) Three enzymes (UGP3, SQD1 and SQD2) are involved in the biosynthesis of SQDG in the chloroplasts of Arabidopsis . SQD2 is responsible for SQDG synthesis under P-sufficient conditions. Under P-deficient conditions, SQD2 produces not only SQDG but also GlcADG. ( b ) Wild-type plants and a series of SQDG-deficient mutants of A. thaliana grown under P-sufficient conditions were transferred to either P-sufficient or P-depleted medium. After cultivation for 4 weeks, the growth of each genotype was compared. The individuals showing the most typical phenotype of P deprivation are displayed. Only 2 sqd2 mutants appeared bleached under P-starvation conditions. Scale bar, 1 cm. Images of other individuals are shown in Supplementary Fig. S11 . Full size image GlcADG deficiency leads to significant growth defects An Arabidopsis mutant with disrupted SQD2 demonstrates impaired growth in the P-limited condition [12] . Therefore, we carefully examined the lipid profiles and growth of a series of SQDG-deficient Arabidopsis mutants with identical genetic backgrounds. Under the P-sufficient condition, the total levels of PG were slightly higher in the SQDG-deficient mutants than in the wild-type ( Fig. 3b ), as previously reported [11] , [12] , [17] . Detailed analysis revealed that 34:2–34:4 PG and 34:3 PI accumulated more in the SQDG-deficient mutants than in the wild-type ( Supplementary Fig. S8 ). Upon P limitation, the ugp3 and sqd1 mutants accumulated GlcADG at slightly higher levels than the wild-type ( Fig. 3b and Supplementary Fig. S9 ). In addition, the decrease of PI, PG and PE following P limitation was suppressed in the SQDG-deficient mutants, as the total levels of GlcADG and SQDG were lower ( Fig. 3b ). In particular, 34:2–34:3 PI and 34:2–34:3 and 36:5 PE were significantly elevated in the sqd2 mutant compared with the other tested genotypes ( Supplementary Fig. S9 ). In contrast to these significant changes in phospholipids, the deficiency of GlcADG and SQDG led to only a subtle effect on galactolipid (MGDG and DGDG) contents ( Fig. 3b ). The levels of glucosylceramide (GlcCer) and steryl glucoside (StGlc), which serve along with glycerolipids as membrane lipids, were also analysed. The amount of GlcCer and StGlc increased following P limitation, and the amounts of StGlc in P-starved sqd2 was higher compared with the other tested genotypes ( Supplementary Fig. S10ab ). There were no clear differences in the total levels of GlcCer among the tested genotypes when P starved, although there were some differences among their GlcCer profiles ( Supplementary Fig. S10c ). These results indicate that the lipid remodelling mechanisms induced by P limitation are significantly altered by GlcADG deficiency. We then investigated the growth of the SQDG-deficient mutants under P-depleted conditions. Under P-sufficient conditions, all SQDG-deficient mutants and the wild-type demonstrated similar growth ( Supplementary Fig. S11a ). In contrast, under P-depleted conditions, the two independent sqd2 mutants that did not accumulate SQDG or GlcADG were severely damaged compared with the sqd1 and ugp3 mutants, in which SQDG is absent but GlcADG is still produced ( Fig. 4b and Supplementary Fig. S11b ). These results indicate that GlcADG has a major role in mitigating P-depletion stress in plants. In addition, the leaf colour of the P-starved sqd2 mutants appeared bleached. The total chlorophyll content was reduced in sqd2 mutants compared with wild-type, ugp3 or sqd1 when plants were grown under P depletion ( Supplementary Fig. S12 ). These results indicate that GlcADG deficiency accelerates the breakdown of chlorophylls and the de-regulation of chloroplast functions. As described above, the disruption of the SQD2 gene in Arabidopsis led to the de-regulation of lipid remodelling under P depletion, and the shoots of sqd2 mutants showed enhanced senescence compared with other SQDG-deficient mutants. These data suggest that P i levels might be affected by disruption of SQD2 . Thus, we analysed the inorganic P i level in shoots grown under P-controlled conditions. The inorganic P i levels in shoots were significantly altered as P i availability changed, whereas there was no significant difference in the P i content of the shoots of the tested genotypes ( Supplementary Fig. S13 ). Thus, the severe growth defects observed in the shoots of sqd2 mutants under P-limited conditions are not necessarily related to the free P i content in shoots, suggesting an association of GlcADG in the protection of the membrane environment under P-limited growth conditions. To obtain further insight into the general role of GlcADG in P depletion in plants, the distribution of GlcADG was also investigated in rice ( Oryza sativa L.). GlcADG was detected in the leaves of rice grown even under the nutrition-sufficient condition ( Supplementary Fig. S14 ), and the levels were significantly elevated (5–7 times) by P deprivation, as observed in A. thaliana ( Fig. 5 ). Significant lipid profile changes upon P limitation were also observed in rice leaves, as observed in A. thaliana ( Supplementary Fig. S15 ). These results suggest a general physiological significance for this novel lipid under P-limited conditions across plant species. 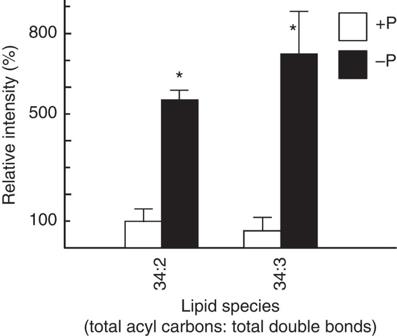Figure 5: GlcADG inducibly accumulates in rice leaves upon P limitation. Comparison of GlcADG levels in the leaves of rice grown under either P-sufficient (+P) or P-depleted (−P) conditions. The levels of each lipid molecule are expressed as relative values compared with the level of 34:2 GlcADG in rice grown under P-sufficient growth conditions. Each data point represents the mean value of three experiments ±s.d. Asterisks indicate a statistically significant difference from the P-sufficient growth condition (*P<0.05, Welch’st-test). More detailed data can be found inSupplementary Figs S14, S15. Figure 5: GlcADG inducibly accumulates in rice leaves upon P limitation. Comparison of GlcADG levels in the leaves of rice grown under either P-sufficient (+P) or P-depleted (−P) conditions. The levels of each lipid molecule are expressed as relative values compared with the level of 34:2 GlcADG in rice grown under P-sufficient growth conditions. Each data point represents the mean value of three experiments ±s.d. Asterisks indicate a statistically significant difference from the P-sufficient growth condition (* P <0.05, Welch’s t -test). More detailed data can be found in Supplementary Figs S14, S15 . Full size image SQDG is an unusual glycerolipid because its polar headgroup consists of SQ, a 6-deoxy-6-sulfonate-glucose ( Fig. 4 ). Much has been speculated about the possible function of this lipid in plants [41] . However, the isolation of SQDG-deficient bacterial mutants [42] , [43] , a mutant of the unicellular algae Chlamydomonas [44] , and a mutant of the plant A. thaliana [12] have all provided some clues about its function. It has become apparent from these mutants that there is no essential role for SQDG in photosynthetic bacteria or in eukaryotic cells containing chloroplasts because all mutants are capable of photoautotrophic growth. The effects on photosynthesis are subtle under normal growth conditions. However, if these SQDG-deficient null mutants are starved for P, they cease growth much earlier than the corresponding wild-type [12] , [42] , [43] . Thus, SQDG has been considered to be of conditional importance in these organisms, including plants. In addition, SQDG and PG contents are known to be maintained by reciprocally balancing their levels with changes in P availability, which is considered to contribute to the maintenance of the negative charge in thylakoid membranes [12] , [45] . However, among the three SQDG-deficient mutants of A. thaliana , the severe growth defect under the P-limited condition was observed only in the sqd2 mutant ( Fig. 4b and Supplementary Fig. S11 ) [12] , and no studies have investigated the differences in the lipid profiles of these SQDG-deficient mutants [11] , [12] , [17] . Our present results unexpectedly revealed that the P-starved sqd2 mutant of A. thaliana lacks not only SQDG but also a novel anionic glycolipid GlcADG, which results in a severe phenotype in this mutant that is not observed in the other two SQDG-deficient mutants analysed in this study. In addition, under P limitation, the ugp3 and sqd1 mutants accumulated slightly higher levels of GlcADG than the wild-type and showed no apparent growth defects. These results collectively indicate the following: (1) GlcADG is a novel molecule importantly involved in the protection against P-depletion stress in plants; (2) the growth defect of P-starved sqd2 is attributable to the deficiency of the two anionic glycolipids SQDG and GlcADG; and (3) moderate increases in GlcADG can compensate for the SQDG deficiency, as shown in the sqd1 and ugp3 mutants. Our results reinforce the importance of plant SQDG synthase and anionic glycolipids synthesized by SQDG synthase during growth under P-limited conditions. The details of the biosynthesis of GlcADG remain unknown except for the fact that SQDG synthase is required for GlcADG biosynthesis. We propose a possible biosynthetic scheme for this glycolipid in Fig. 4 . However, our lipidomic data using a few SQDG-deficient mutants do not deny the possibility of interconversion of SQDG and GlcADG. Other types of experiments, such as flux analysis, will be important in understanding the metabolic flow underlying the accumulation of these two anionic glycolipids. It is also postulated that the inducible synthesis of GlcADG under P starvation entails increased synthesis of an unidentified sugar donor, presumably UDP-GlcA, in chloroplasts. Our current study suggests the possibility of the presence of an uncharacterized biosynthetic pathway or transportation mechanism for UDP-GlcA in chloroplasts. The synthesis of GlcADG by dehydrogenation of monoglucosyldiacylglycerol, found in several plants [46] , is also possible. In P-starved sqd2 mutants, the levels of PI and PE were significantly elevated, which indicates that the complete deficiency of anionic glycolipids causes the de-regulation of not only PG but also other phospholipids, such as PI and PE. Thus, levels of these phospholipids (PI and PE) and GlcADG are also reciprocally maintained in plant cells under P-limited conditions ( Fig. 6 ), as a similar relationship can be found between SQDG and PG, suggesting some shared functions among GlcADG, PI and PE under P-limited conditions. Levels of 34:3 PI and 34:3 PE were also slightly elevated in sqd1 and ugp3 mutants compared with wild-type even under P sufficiency ( Supplementary Fig. S8 ). Thus, these phospholipids may also generally contribute to the maintenance of proper membrane properties in plants even under P sufficiency, and their roles may become more important when plants are deficient in two anionic glycolipids under P-depleted conditions. 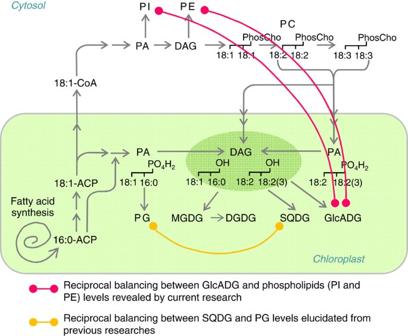Figure 6: Anionic glycolipids and phospholipids are reciprocally balanced under P depletion. An abbreviated biosynthetic scheme for the major plant polar glycerolipids is represented along with the results of the current report. Previous research on several SQDG-deficient mutants suggested that the levels of SQDG and PG are reciprocally regulated (orange line), while our current report suggests that a similar reciprocal regulation also can be found among GlcADG, PI and PE (red lines). The levels of SQDG, PI and PE might also be reciprocally maintained. Figure 6: Anionic glycolipids and phospholipids are reciprocally balanced under P depletion. An abbreviated biosynthetic scheme for the major plant polar glycerolipids is represented along with the results of the current report. Previous research on several SQDG-deficient mutants suggested that the levels of SQDG and PG are reciprocally regulated (orange line), while our current report suggests that a similar reciprocal regulation also can be found among GlcADG, PI and PE (red lines). The levels of SQDG, PI and PE might also be reciprocally maintained. Full size image Currently, contributions to the compensation of the deficiency of anionic glycolipids are likely to be significant in the order of PG>PI>PE, although it remains unknown whether this order is because of the difference in chemical properties or the difference in the organelle where they are mainly synthesized, that is, chloroplastic PG is synthesized in chloroplasts [47] , such as SQDG and presumably GlcADG, whereas PI and PE are mainly synthesized in the endoplasmic reticulum ( Fig. 6 ). We have never determined where GlcADG is synthesized and accumulates, but GlcADG is likely synthesized in chloroplasts because SQDG synthase is localized in the chloroplast inner membrane [37] . The idea that GlcADG accumulates in chloroplasts is plausible considering the localization of SQDG synthase, although we cannot exclude the possibility that somehow GlcADG is exported from chloroplasts to extraplastidic membranes such as DGDG [6] , [8] . Given that GlcADG accumulates in extraplastidic space, we might be able to determine the reason why the levels of GlcADG, PI and PE are reciprocally regulated in P-starved plants. In addition, we cannot deny the possibility that levels of PI and PE in the chloroplast membrane are elevated in sqd2 mutants under P deficiency even though PE is usually not abundant in chloroplasts [48] . Further research to determine the localization of GlcADG accumulation will help us to understand this phenomenon. A study on the bacterium B. diminuta also investigated the replacement of acidic phospholipids by GlcADG upon P limitation [49] , suggesting a functional convergence of lipid remodelling involving the accumulation of GlcADG across kingdoms. No information regarding the genes involved in GlcADG biosynthesis in B. diminuta is currently available. Lipid remodelling in membrane systems under P-limited conditions is considered to contribute to sustaining the level of cellular inorganic P i by modifying the P allocation in the cell. As described above, lipid remodelling is severely de-regulated in a P-starved sqd2 mutant, but there is no significant decrease in free P i in this mutant ( Supplementary Fig. S13 ). These results suggest that GlcADG is not essential to maintain the free P i level in P-starved plants but that it is likely to contribute to the control of the membrane environment to ensure the proper functioning of organelles, including chloroplasts, in P-limited, unfavourable environments. In addition, this study suggests that plants have developed an alternative mechanism to maintain a negative membrane charge by synthesizing uronic acid-containing lipids free of sulphur, which is also an essential macronutrient requiring significant energy for its assimilation [50] . Genome sequence information on organisms capable of synthesizing SQDG has revealed that the two genes coding UDP-SQ synthase and SQDG synthase evolved at different times, and while many genomes show readily identifiable UDP-SQ synthase orthologs, SQDG synthases were differently recruited in cyanobacteria/plants versus non-cyanobacteria and archaea [51] . The involvement of plant SQDG synthase in different anionic glycolipids might be related to its ancestral function, which might still be retained in plants to allow them adapt to unfavourable surroundings. Chemicals Primuline, (trimethylsilyl)diazomethane (2.0 M in diethyl ether), and 1,2-didecanoyl-sn-glycero-3-phosphocholine were obtained from Sigma-Aldrich, and polypropylene glycol 2000 (PPG-2000) was obtained from Alfa Aesar. Glucuronic acid was purchased from Tokyo Chemical Industry. Unless stated otherwise, all other chemicals were purchased from Wako Pure Chemical Industries. Nuclear magnetic resonance 1 H NMR spectra were recorded in CDCl 3 supplemented with a drop of D 2 O for H-D exchange. Other NMR spectra ( 13 C, COSY, HMQC, HMBC and DEPT) were recorded in absolute CDCl 3 . Tetramethylsilane was used for the internal standard. Plant materials A. thaliana —Seeds of T-DNA insertion lines for sqd2-1 (SALK_070595) and sqd2-2 (SALK_139798) were purchased from ABRC at Ohio State University [52] . The T-DNA insertion sites of these lines were confirmed by sequencing PCR fragments ( Supplementary Fig. S16 ). A PCR fragment at the left border of the T-DNA of sqd2-1 was amplified using LBa1 and SALK_070595_Fw , and the right border of the T-DNA of sqd2-2 was amplified using SALK_070595_Fw and RBa1 ( Supplementary Table S1 ). The sqd1 , ugp3-1 and ugp3-2 mutants were isolated in our previous study based on the results of genome PCR [17] and used again in this research. Seeds of the sqd2 mutant in the Ws-0 background (provisionally named sqd2-3 in this study) and its wild-type were kind gifts from Professor Benning [12] . Surface-sterilized seeds were sown on agar-solidified Murashige and Skoog medium [53] containing 1% (w/v) sucrose at 22 °C under 16 h light/8 h dark cycles. Photon flux density was 50 μmol m –2 sec –1 . The seedlings were kept on agar for 14 days before transfer to plates with controlled phosphate (P i ) concentrations. For P-limitation experiments, sterile Arabidopsis medium [54] was used but at half concentration and containing 0.8% (w/v) agar, 20 mM MES (pH 6.0) and different concentrations of KH 2 PO 4 as indicated [7] . For lipid analysis, leaves were harvested 6 h after the onset of the light phase, frozen in liquid nitrogen and stored at −80 °C until lipid extraction. Rice—Dehulled seeds of O. sativa L. cv. Nipponbare were sterilized and germinated on agar-solidified Murashige and Skoog medium at 28 °C under a 16 h light/8 h dark cycle. To expose plants to P-limiting stress, 5-day-old seedlings were transplanted and hydroponically cultured in the P-controlled medium used for the stress treatment of A. thaliana . The culture medium was changed every week. Lipidomics by HILIC-MS Plant lipids were extracted following the method of Bligh and Dyer [55] with slight modifications [26] , and directly subjecting the extract to LC-MS analysis. The lipidomic data were recorded on an LC-MS-IT-TOF mass spectrometer using electrospray ionization, combined with an LC-20AD HPLC system (Shimadzu) [26] . Parameters for MS were as follows: scan range, m/z 150–1,600; loop time, 0.6 s; CDL and heat block temperature, 160 °C; nebulizer gas (N 2 ), 1.5 l min –1 . More details are found in our previous report [26] and metadata in ‘ Supplementary Data Set.xls’. Peak picking and alignment were performed using the Profiling Solution software (version 1.0.76.0; Shimadzu). The profiling solution parameters were as follows: ion m/z tolerance, 20 mDa; ion RT tolerance, 0.1 min; ion intensity threshold, 2e4; detect isomer valley, 20%; allow some ion without isotope peak, ON [26] . The data matrix containing ~480 ions consisting of negatively detected ions was exported from the profiling solution software and normalized relative to the intensity of the [M+HCO 2 ] − ion of the internal standard (1,2-didecanoyl-glycero-3-phosphocholine). Annotation was based on the theoretical m/z values of each lipid species and the retention time of identified compounds with the same polar head [26] . Statistics for the analysis of lipidomic data Normalized LC-MS data were pareto-scaled and subjected to OPLS-DA using SIMCA-P (version 11.0.0.0; Umetrics). Tukey’s test and Welch’s t -test were performed using their respective functions (TukeyHSD and t -test) in the statistical software R version 2.14.0 ( http://www.r-project.org/ ). HCL and jackknife testing were performed on MultiExperiment Viewer (MeV) version 4.8 ( http://www.tm4.org/mev/ ). For HCL, Pearson’s correlations were used to analyse the distance metric. Average linkage clustering was selected for the linkage method. The data set used for HCL is available as ‘ Supplementary Data Set.xls’. Metadata also can be found in the same file. Preparation of GlcADG from A. thaliana and B. diminuta A. thaliana plants (Col-0 accession, 340 g fresh weight) grown under P deficiency as described above were extracted using the same protocol to prepare samples for lipidomic analysis. The resulting lipid extracts (4.1 g) was loaded onto a silica gel column (silica gel 60 N, spherical, neutral; 25-cm long, 7-cm i.d. ; Kanto Chemical) equilibrated with chloroform. The column was washed with chloroform (3 l), chloroform–acetone (1:1, v/v, 3.6 l), acetone (1 l), acetone–methanol (1:1, v/v, 1 l) and methanol (1 l). The acetone–methanol fractions containing UK1 were subjected to preparative thin-layer chromatography on Silica Gel 60 plates containing no fluorescent indicator (Merck) using chloroform–methanol–H 2 O (65:25:4, v/v/v). After spraying a primuline solution, lipids were detected under UV light. The fluorescent spots containing UK1 were scraped off and further subjected to preparative thin-layer chromatography with a chloroform–methanol–acetic acid solution (75:25:3, v/v/v) to obtain UK1 ( 1 , 9.6 mg). MS/MS of all detectable UK1 molecules, are found in Fig. 2 and Supplementary Figs S2,S3 . B. diminuta ATCC 11568 (Strain JCM 2788) was provided by RIKEN BRC (Wako, Japan). The strain was rehydrated according to the provider’s instructions and cultivated with continuous rotation at 180 r.p.m. in lysogeny broth containing PPG-2000 (50 p.p.m.) as antifoam. After a 48-h incubation at 30 °C, the cells were collected by centrifugation. The dried cells (4.43 g) were extracted with mixtures of chloroform, methanol and diethyl ether to yield crude lipid extracts (320 mg) as previously reported [56] , [57] . The extracts were separated to purify GlcADG (17.8 mg) using the same protocol described above for the purification of UK1. MS and MS/MS of the bacterial GlcADG are found in Supplementary Fig. S4 . Preparation of the methyl ester of GlcADG GlcADG from B. diminuta and UK1 from A. thaliana were methylated with (trimethylsilyl)diazomethane as previously described [58] . The 1 H and 13 C NMR spectra and key HMBCs of bacterial GlcADG are shown in Supplementary Figs S17–S19 . Methyl ester of GlcADG from B. diminuta. 1 H NMR (500 MHz, CDCl 3 ) δ 0.84–0.93 (6 H, m , –CH 2 C H 3 ), 1.19–1.45(ca 36 H, m , –CH 2 –), 1.54–1.66 (4 H, m , –OCOCH 2 C H 2 –), 1.93––2.10 (5 H, m , –CH=CHC H 2 –), 2.25–2.39 (4 H, m , –OCOC H 2 R), 3.57 (1 H, dd , J =3.7, 9.5 Hz, H-2′), 3.67 (1 H, dd , J =5.7, 10.9 Hz, H-3a), 3.72 (1 H, triplet-like dd , J =8.9, 9.5 Hz, H-4′), 3.78 (1 H, triplet-like dd , J =8.9, 9.5 Hz, H-3′), 3.83 (3 H, s , CH 3 O-6′), 3.90 (1 H, dd , J =4.6, 10.9 Hz, H-3b), 4.15 (1 H, dd , J =5.7, 11.9 Hz, H-1a), 4.16 (1 H, d , J =9.5 Hz, H-5′), 4.41 (1 H, dd , J =4.2, 11.9 Hz, H-1b), 4.94 (1 H, d , J =3.7 Hz, H-1′), 5.26 (1 H, m , H-2), 5.33–5.36 (2 H, m , –CH=CH–); 13 C NMR (125 MHz, CDCl 3 ) δ 14.1 (–CH 2 C H 3 ), 22.66–22.70 (–CH 2 C H 2 CH 3 ), 24.9 (–OCOCH 2 C H 2 CH 2 –), 27.2 (–CH=CH C H 2 CH 2 –), 28.7–31.9 (–CH 2 C H 2 CH 2 –), 34.1–34.2 (–OCO C H 2 CH 2 –), 52.9 ( C H 3 O-6′), 61.9 (C-1), 67.1 (C-3), 69.6 (C-2), 70.6 (C-5′), 71.5 (C-2′, C-4′), 73.6 (C-3′), 99.1 (C-1′), 129.8 (–CH=CH–), 130.0 (–CH=CH–), 170.5 (C6′), 173.2 (–O C OR of fatty acid), 173.5 (–O C OR of fatty acid). Methyl ester of UK1 from A. thaliana. 1 H NMR (500 MHz, CDCl 3 ) δ 0.85–0.93 (ca 4 H, m , –CH 2 C H 3 ), 0.95–1.02 (ca 3 H, –CH=CHCH 2 C H 3 ), 1.2–1.4 (ca 40 H, m , –CH 2 –), 1.5–1.7 (ca 13 H, m , –OCOCH 2 C H 2 –), 2.01–2.13 (ca 6 H, m , –CH=CHC H 2 –), 2.27–2.37 (ca 4 H, m , –OCOC H 2 R), 2.74–2.84 (ca 4 H, m , –CH=CHC H 2 CH=CH–), 3.58 (1 H, dd , J =3.7, 9.5 Hz, H-2′), 3.68 (1 H, dd , J =5.7, 10.9 Hz, H-3a), 3.72 (1 H, triplet-like dd , J =8.9, 9.5 Hz, H-4′), 3.79 (1 H, triplet-like dd , J =8.9, 9.5 Hz, H-3′), 3.84 (3 H, s , CH 3 O-6′), 3.91 (1 H, dd , J =4.6, 10.9 Hz, H-3b), 4.14 (1 H, dd , J =5.7, 12.0 Hz, H-1a), 4.17 (1 H, d , J =9.5 Hz, H-5′), 4.42 (1 H, dd , J =4.3, 12.0 Hz, H-1b), 4.95 (1 H, d , J =3.7 Hz, H-1′), 5.23–5.29 (ca 1 H, m , H-2), 5.29–5.44 (ca 8 H, m , -CH=CH-); 13 C NMR (125 MHz, CDCl 3 ) δ 14.06–14.3 (-CH 2 C H 3 ), 20.5 (-CH=CH C H 2 CH 3 ), 22.6–22.7 (-CH 2 C H 2 CH 3 ), 24.8 (-OCOCH 2 C H 2 CH 2 -), 25.5–25.6 (-CH=CH C H 2 CH=CH-), 27.2 (-CH=CH C H 2 CH 2 -), 29.1–31.9 (-CH 2 C H 2 CH 2 -), 34.1–34.2 (-OCO C H 2 CH 2 -), 52.8 ( C H 3 O-6′), 61.9 (C-1), 67.1 (C-3), 69.7 (C-2), 70.6 (C-5′), 71.5 (C-2′, C-4′), 73.6 (C-3′), 99.1 (C-1′), 127.1–132.0 (olefinic carbons of fatty acids), 170.4 (C6′), 173.1 (-O C OR of fatty acid), 173.5 (-O C OR of fatty acid). Quantification of inorganic P i in plants Leaves (30 mg) were frozen in liquid nitrogen and homogenized using a Mixer Mill MM300 (Retsch, Haan, Germany) for 2 min at 15 Hz with a zirconium bead and then extracted with 50% (v/v) aqueous methanol (300 μl) followed by centrifugation at 12,000 g . The milling process was carried out under cryogenic conditions (the grinding jars were cooled with liquid nitrogen before each milling process to ensure a low milling temperature and keep the plants frozen). The measurement of P i content in the supernatants was accomplished by forming a phosphomolybdate complex and in turn reducing it to a molybdenum blue complex [59] . How to cite this article: Okazaki, Y. et al. A new class of plant lipid is essential for protection against phosphorus depletion. Nat. Commun. 4:1510 doi: 10.1038/ncomms2512 (2013).